Root-derived CLE glycopeptides control nodulation by direct binding to HAR1 receptor kinase Leguminous plants establish a symbiosis with rhizobia to enable nitrogen fixation in root nodules under the control of the presumed root-to-shoot-to-root negative feedback called autoregulation of nodulation. In Lotus japonicus , autoregulation is mediated by CLE-RS genes that are specifically expressed in the root, and the receptor kinase HAR1 that functions in the shoot. However, the mature functional structures of CLE-RS gene products and the molecular nature of CLE-RS/HAR1 signalling governed by these spatially distant components remain elusive. Here we show that CLE-RS2 is a post-translationally arabinosylated glycopeptide derived from the CLE domain. Chemically synthesized CLE-RS glycopeptides cause significant suppression of nodulation and directly bind to HAR1 in an arabinose-chain and sequence-dependent manner. In addition, CLE-RS2 glycopeptide specifically produced in the root is found in xylem sap collected from the shoot. We propose that CLE-RS glycopeptides are the long sought mobile signals responsible for the initial step of autoregulation of nodulation. Many leguminous plant species establish a symbiotic association with rhizobia that induces the formation of nodules on roots. This symbiosis enables nitrogen fixation in the nodules and is beneficial to the host plants; however, excessive nodule formation is deleterious to the plants because the energy cost outweighs the need for fixed nitrogen. To achieve a balance in this symbiotic relationship, the host plant tightly controls the number of nodules via a root-to-shoot-to-root negative feedback signalling loop commonly termed autoregulation of nodulation [1] , [2] , [3] , [4] . The initial step of autoregulation is thought to involve long-distance signalling from the root to the shoot [5] , [6] , [7] . This hypothesis was strongly supported by the findings from analyses of the Lotus japonicus hypernodulating mutant, hypernodulation aberrant root formation ( har1 ) [8] , [9] , [10] , and orthologous mutants in other leguminous species [8] , [9] , [11] , [12] . HAR1 encodes a leucine-rich repeat receptor kinase (LRR-RK) that is expressed in both roots and shoots [8] , [9] . Grafting experiments showed that HAR1 in the shoot is required to control nodule number in the root. Thus, HAR1 has been suggested to function in the shoot as a receptor for a signal emanating from the roots. HAR1 has high similarity to Arabidopsis CLAVATA1 (CLV1) [13] , a protein known to act as a receptor for the shoot apical meristem regulator CLV3 of the CLV3/ESR-related (CLE) small secreted peptide family [14] , [15] . A search for L. japonicus CLE family genes involved in nodulation identified two genes, CLE-RS1 and CLE-RS2 that are highly upregulated in roots that have been inoculated with rhizobia [16] . Overexpression of these CLE genes in hairy roots resulted in the systemic inhibition of nodulation in a HAR1-dependent manner. CLE-RS2 is also strongly upregulated in the roots of plants grown under high nitrate conditions that are known to abolish nodulation. Conversely, knockdown of Medicago truncatula MtCLE12 and MtCLE13 resulted in a significant increase in nodule number [17] . Functionally similar CLE genes have also been identified in other leguminous species [18] , [19] , [20] , [21] . Thus, CLE-RS peptides are strong candidates for the root-derived signals that might act as ligands for HAR1. However, commercially synthesized CLE-RS peptides did not suppress nodulation [16] , suggesting that some specific modifications are required for the activity of CLE-RS peptides. Furthermore, the molecular basis of a CLE-RS/HAR1 signalling that involves such spatially distant components remains elusive. In the present study, we used biochemical approaches to explore the bioactive forms of CLE-RS peptides and to identify their modes of action in long-distance regulation of nodulation. We found that arabinosylated CLE-RS peptides suppress nodulation and directly bind to HAR1 receptor kinase. Furthermore, we show that CLE-RS2 glycopeptide can travel from the roots to the shoot. These findings suggest that the CLE-RS peptides mediate organ-to-organ communication. CLE-RS2 is an arabinosylated glycopeptide Secreted peptides involved in signalling pathways in plants often undergo post-translational modification and proteolytic processing that alter their biological functions and specific receptor interactions [22] , [23] . To determine the mature functional structure of CLE-RS peptides, we used a whole-plant submerged-culture system to analyse secreted peptides that had accumulated in the apoplast of Arabidopsis plants overexpressing CLE-RS2 . Under submerged-culture conditions, any secreted peptides in the apoplast diffuse directly into the culture medium [24] . Nano-liquid chromatography mass spectrometry (nano-LC-MS) and nano-liquid chromatography tandem mass spectrometry (nano-LC-MS/MS) analyses of peptides that diffused from the apoplast identified a peak that eluted at 34.9 min ( m / z 908.9 [M+2H] 2+ and m/z 606.3 [M+3H] 3+ ); this peak represents the mature 13-amino-acid CLE-RS2 peptide that is derived from the C-terminal region of the precursor polypeptide ( Fig. 1a–c ). Notably, the seventh hydroxyproline (Hyp 7 ) residue of this peptide is post-translationally modified with three residues of arabinose ( Fig. 1d ). 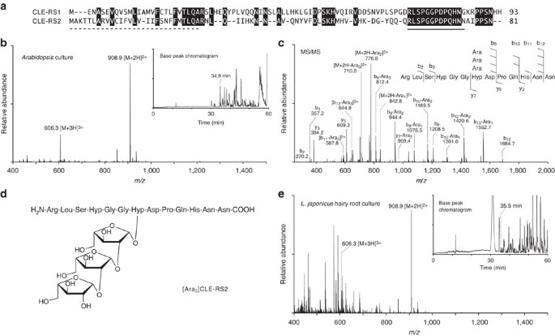Figure 1: Structural elucidation of mature CLE-RS2 peptide. (a) Amino-acid sequence alignment of the polypeptides encoded byCLE-RS1andCLE-RS2. Mature [Ara3]CLE-RS2 peptide-derived region is underlined, and the predicted secretion signal peptide is indicated by dashed line. The conserved region is shaded in black. (b) Detection of mature CLE-RS2 peptide secreted fromArabidopsisplants overexpressingCLE-RS2at 34.9 min. Inset shows nano-LC-MS base peak chromatogram. (c) Nano-LC-MS/MS spectrum for the mature CLE-RS2 peptide. (d) Structure of the mature CLE-RS2 peptide ([Ara3]CLE-RS2). (e) Detection of mature CLE-RS2 peptide secreted byL. japonicushairy roots overexpressingCLE-RS2at 35.5 min. Inset shows nano-LC-MS base peak chromatogram. Figure 1: Structural elucidation of mature CLE-RS2 peptide. ( a ) Amino-acid sequence alignment of the polypeptides encoded by CLE-RS1 and CLE-RS2 . Mature [Ara 3 ]CLE-RS2 peptide-derived region is underlined, and the predicted secretion signal peptide is indicated by dashed line. The conserved region is shaded in black. ( b ) Detection of mature CLE-RS2 peptide secreted from Arabidopsis plants overexpressing CLE-RS2 at 34.9 min. Inset shows nano-LC-MS base peak chromatogram. ( c ) Nano-LC-MS/MS spectrum for the mature CLE-RS2 peptide. ( d ) Structure of the mature CLE-RS2 peptide ([Ara 3 ]CLE-RS2). ( e ) Detection of mature CLE-RS2 peptide secreted by L. japonicus hairy roots overexpressing CLE-RS2 at 35.5 min. Inset shows nano-LC-MS base peak chromatogram. Full size image To determine whether the mature peptide structure of CLE-RS2 in L. japonicus is identical to that in Arabidopsis , we used Agrobacterium -mediated hairy root transformation to overexpress CLE-RS2 in L. japonicus ; the secreted peptides that accumulated in the hairy root submerged-culture medium were analysed by nano-LC-MS and nano-LC-MS/MS. We detected a peak of m / z 908.9 and m/z 606.3 at 35.5 min that corresponds to the 13-amino-acid arabinosylated CLE-RS2 peptide ( Fig. 1e ). The MS/MS spectrum of this peak showed a fragmentation pattern identical to that of Arabidopsis, indicating that CLE-RS2 is also arabinosylated in L. japonicus ( Supplementary Fig. S1 ). We concluded that the mature form of CLE-RS2 is a 13-amino-acid glycopeptide in which the Hyp 7 residue is post-translationally modified with three residues of arabinose. Hereafter, we refer to this glycopeptide as [Ara 3 ]CLE-RS2. Chemical synthesis of [Ara 3 ]CLE-RS glycopeptides Modification of Hyp residues by arabinose is a plant-specific post-translational modification of peptides synthesized through secretory pathways [25] , [26] . A previous analysis of triarabinoside structures on the Arabidopsis CLV3 peptide showed that the Hyp residue was modified by three L -arabinose moieties with a linear β-1,2-linkage [26] . As [Ara 3 ]CLE-RS2 is present in plants at too low a level to obtain sufficient quantities for functional analyses, we decided to chemically synthesize [Ara 3 ]CLE-RS2. We based our synthesis on the method recently described for stereoselective synthesis of arabinosylated CLV3 in Arabidopsis [27] . In brief, a chemically synthesized triarabinosylated Hyp building block was incorporated into the peptide-resin at position Hyp 7 using solid-phase peptide synthesis. After acidolytic release from the resin, the crude glycopeptide was deacetylated and purified by high-performance liquid chromatography (HPLC) to yield analytically pure [Ara 3 ]CLE-RS2. We confirmed that the retention time and MS/MS fragmentation pattern of the synthetic [Ara 3 ]CLE-RS2 were identical to those of natural [Ara 3 ]CLE-RS2 ( Supplementary Fig. S2 ). We also prepared 13-amino-acid [Ara 3 ]CLE-RS1 glycopeptide based on the sequence similarity of the conserved mature peptide domain. [Ara 3 ]CLE-RS glycopeptides suppress nodulation To test whether [Ara 3 ]CLE-RS2 could act as a signal to negatively regulate nodulation, we applied various concentrations of synthetic [Ara 3 ]CLE-RS2 to L. japonicus seedlings. As HAR1 in the shoot is involved in the control of nodule number in the root, we applied the [Ara 3 ]CLE-RS2 solution directly to the shoot by cutting the surface of the cotyledons. We visually confirmed successful uptake by the appearance of a blue dye marker in the primary leaves of the shoot ( Supplementary Fig. S3 ). In wild-type plants, concentrations of [Ara 3 ]CLE-RS2 as low as 100 nM suppressed nodulation without altering root growth ( Fig. 2a,b and Supplementary Fig. S4 ). By contrast, neither non-arabinosylated CLE-RS2 peptide (CLE-RS2p) nor Arabidopsis arabinosylated CLV3 peptide ([Ara 3 ]CLV3) showed any effect on nodulation ( Fig. 2a–c ), indicating that both the arabinose chain and the backbone peptide sequence are critical to the function of [Ara 3 ]CLE-RS2. We also confirmed that synthetic [Ara 3 ]CLE-RS1 glycopeptide could suppress nodulation in a similar dose-dependent manner as [Ara 3 ]CLE-RS2 ( Fig. 2d ). 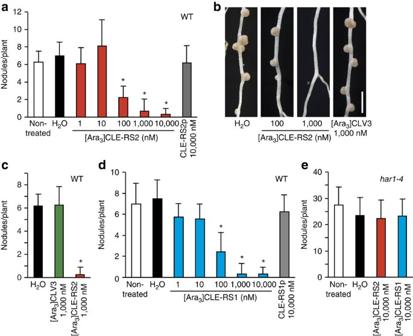Figure 2: Synthetic [Ara3]CLE-RS peptides suppress nodulation. (a) Effect of synthetic [Ara3]CLE-RS2 on nodule formation in wild-type (WT) plants (n=8–14). [Ara3]CLE-RS2 was applied to the plants via a cut in the surface of the cotyledon. The number of nodules was counted 15 days after peptide application. (b) Nodules formed in roots of wild-type plants with or without application of [Ara3]CLE-RS2 or [Ara3]CLV3. Photographs were taken 14 days after inoculation with rhizobia. Scale bars, 2 mm. (c) Effect of [Ara3]CLV3 peptide on nodule formation in wild-type plants (n=12). (d) Effect of synthetic [Ara3]CLE-RS1 on nodule formation in wild-type plants (n=8–14). (e) Effect of [Ara3]CLE-RS2 and [Ara3]CLE-RS1 on nodule formation inhar1-4mutant plants (n=9–16). (a,c–e) Error bar indicates mean±s.d. Statistical differences were evaluated using at-test. Statistically significant differences (P<0.01) compared with H2O-applied plants are indicated by asterisk. Figure 2: Synthetic [Ara 3 ]CLE-RS peptides suppress nodulation. ( a ) Effect of synthetic [Ara 3 ]CLE-RS2 on nodule formation in wild-type (WT) plants ( n =8–14). [Ara 3 ]CLE-RS2 was applied to the plants via a cut in the surface of the cotyledon. The number of nodules was counted 15 days after peptide application. ( b ) Nodules formed in roots of wild-type plants with or without application of [Ara 3 ]CLE-RS2 or [Ara 3 ]CLV3. Photographs were taken 14 days after inoculation with rhizobia. Scale bars, 2 mm. ( c ) Effect of [Ara 3 ]CLV3 peptide on nodule formation in wild-type plants ( n =12). ( d ) Effect of synthetic [Ara 3 ]CLE-RS1 on nodule formation in wild-type plants ( n =8–14). ( e ) Effect of [Ara 3 ]CLE-RS2 and [Ara 3 ]CLE-RS1 on nodule formation in har1-4 mutant plants ( n =9–16). ( a , c – e ) Error bar indicates mean±s.d. Statistical differences were evaluated using a t -test. Statistically significant differences ( P <0.01) compared with H 2 O-applied plants are indicated by asterisk. Full size image To confirm that the action of CLE-RS peptides is dependent on HAR1, we applied [Ara 3 ]CLE-RS1 and [Ara 3 ]CLE-RS2 to har1-4 mutant plants. The number of nodules on har1-4 mutants was not affected by application of [Ara 3 ]CLE-RS peptides even at 10 μM ( Fig. 2e ). These results indicate that [Ara 3 ]CLE-RS peptides regulate nodule formation via HAR1. [Ara 3 ]CLE-RS glycopeptides directly bind to HAR1 Next, we examined the interaction of [Ara 3 ]CLE-RS peptides with HAR1 using [Ara 3 ]CLE-RS2 derivative tagged with 125 I-labelled photoactivatable 4-azidosalicylic acid ([ 125 I]ASA-[Ara 3 ]CLE-RS2) ( Supplementary Fig. S5 ). Upon treatment with ultraviolet light, the azide group photolyses to form a reactive nitrene, which can form a covalent bond with receptor proteins. Microsomal fractions from tobacco BY-2 cells overexpressing HAR1–HaloTag (HAR1–HT) were photoaffinity labelled with [ 125 I]ASA-[Ara 3 ]CLE-RS2; after SDS–polyacrylamide gel electrophoresis and autoradiography, these fractions showed labelling of a 130-kD band ( Fig. 3a,b ). This band disappeared completely after competitive inhibition by a 300-fold excess of unlabelled [Ara 3 ]CLE-RS2, indicating that [Ara 3 ]CLE-RS2 specifically binds to HAR1. Notably, neither unglycosylated CLE-RS2p nor [Ara 3 ]CLV3 interfered with this binding ( Fig. 3b,d ), indicating that the arabinose chain and the amino acid sequence are critical for [Ara 3 ]CLE-RS2 binding to HAR1. This absolute requirement for arabinose chain and sequence specificity in the receptor interaction explains the results of our nodulation bioassay. [Ara 3 ]CLE-RS1 also effectively competed with [ 125 I]ASA-[Ara 3 ]CLE-RS2 for HAR1 binding in a similar affinity to that of [Ara 3 ]CLE-RS2, confirming that [Ara 3 ]CLE-RS1 also interacts with HAR1 ( Fig. 3c ). 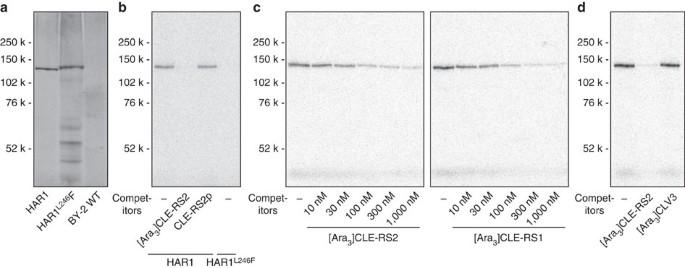Figure 3: [Ara3]CLE-RS peptides directly bind to HAR1. (a) Expression of HAR1–HT and HAR1L246F-HT in transgenic BY-2 cells visualized by specific incorporation of a HaloTag TMR fluorescent dye. HaloTag protein is specifically labelled by HaloTag TMR that contains a haloalkane group. (b) Photoaffinity labelling of HAR1–HT and HAR1L246F-HT with 10 nM [125I]ASA-[Ara3]CLE-RS2 in the absence or presence of 300-fold excess of unlabelled [Ara3]CLE-RS2 or CLE-RS2p. (c) Competitive displacement of [125I]ASA-[Ara3]CLE-RS2 binding to HAR1–HT by various concentrations of unlabelled [Ara3]CLE-RS2 and [Ara3]CLE-RS1. (d) A 300-fold excess of unlabelled [Ara3]CLV3 showed no competitive displacement of [125I]ASA-[Ara3]CLE-RS2 binding to HAR1–HT. Figure 3: [Ara 3 ]CLE-RS peptides directly bind to HAR1. ( a ) Expression of HAR1–HT and HAR1 L246F -HT in transgenic BY-2 cells visualized by specific incorporation of a HaloTag TMR fluorescent dye. HaloTag protein is specifically labelled by HaloTag TMR that contains a haloalkane group. ( b ) Photoaffinity labelling of HAR1–HT and HAR1 L246F -HT with 10 nM [ 125 I]ASA-[Ara 3 ]CLE-RS2 in the absence or presence of 300-fold excess of unlabelled [Ara 3 ]CLE-RS2 or CLE-RS2p. ( c ) Competitive displacement of [ 125 I]ASA-[Ara 3 ]CLE-RS2 binding to HAR1–HT by various concentrations of unlabelled [Ara 3 ]CLE-RS2 and [Ara 3 ]CLE-RS1. ( d ) A 300-fold excess of unlabelled [Ara 3 ]CLV3 showed no competitive displacement of [ 125 I]ASA-[Ara 3 ]CLE-RS2 binding to HAR1–HT. Full size image We tested whether [Ara 3 ]CLE-RS2 could interact with a mutant receptor protein carrying the har1-4 mutation (L246F) [9] . Our analysis showed that [ 125 I]ASA-[Ara 3 ]CLE-RS2 did not bind to the HAR1 L246F –HT mutant receptor ( Fig. 3a,b ). Thus, loss of [Ara 3 ]CLE-RS2 responsiveness in the har1-4 mutant is reflected by a loss of [Ara 3 ]CLE-RS2 binding to HAR1. The har1-4 mutant carries a missense mutation in Leu 246 , which is located within LRR8 and which is known to have a critical role in ligand binding in the CLV1/BAM family receptor kinases in Arabidopsis [28] . We therefore conclude that both [Ara 3 ]CLE-RS1 and [Ara 3 ]CLE-RS2 can function as ligands for HAR1 receptor kinase. [Ara 3 ]CLE-RS2 is transported through the xylem As CLE-RS peptides are exclusively expressed in roots but act through HAR1 in the shoot [8] , [9] , [16] , the results of our ligand binding assay suggested a model in which [Ara 3 ]CLE-RS peptides are translocated from the root to the shoot where they bind to HAR1. As the xylem often mediates the transport of molecules from roots to shoots in higher plants [29] , we hypothesized that [Ara 3 ]CLE-RS peptides might be translocated via the xylem. Because efficient xylem sap collection from L. japonicus is technically difficult, we used the hairy root system in soybean plants that express L. japonicus CLE-RS2 following Agrobacterium -mediated transformation. This transformation system leads to the generation of chimeric plants that have transgenic hairy root systems attached to non-transformed stem and leaves. The shoots of 40-day-old plants were cut at the second internode above the hypocotyl, and xylem sap was then collected for 10 h. The sap was concentrated, partially purified and analysed by nano-LC-MS followed by nano-LC-MS/MS. The selected ion chromatogram for m / z 908.9, which corresponds to [M+2H] 2+ , showed a peak at 34.8 min for xylem sap derived from plants with transgenic hairy roots overexpressing CLE-RS2 ( Fig. 4a ). An MS/MS analysis confirmed that the fragmentation pattern of this peak was identical to that of authentic [Ara 3 ]CLE-RS2 ( Fig. 4c , see also Fig. 1c ). This peak was not detected in xylem sap derived from plants with hairy roots transformed with an empty vector ( Fig. 4b ). 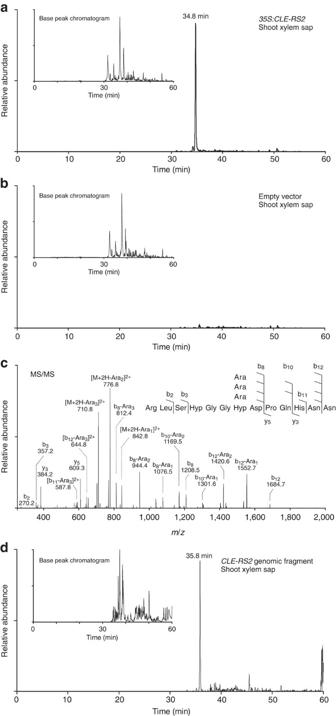Figure 4: Detection of root-derived [Ara3]CLE-RS2 peptide in shoot xylem sap. (a) Nano-LC-MS chromatogram of shoot xylem sap collected from soybean plants, in whichCLE-RS2is overexpressed in transformed hairy roots. Selected ion chromatogram atm/z908.9 that corresponds to [M+2H]2+showed a peak at 34.8 min. Inset shows the base peak chromatogram of shoot xylem sap. (b) Nano-LC-MS chromatogram of shoot xylem sap collected from soybean transformed with an empty vector. Selected ion chromatogram atm/z908.9 indicates the absence of [Ara3]CLE-RS2. (c) MS/MS spectrum of the 34.8 min peak inashowed a fragmentation pattern identical to that of authentic [Ara3]CLE-RS2. (d) Nano-LC-MS chromatogram of shoot xylem sap collected from soybean plants that developed transformed hairy roots after inoculation with a vector harbouring theCLE-RS2genomic region. Selected ion chromatogram atm/z606.3 that corresponds to [M+3H]3+showed a peak at 35.8 min. Inset shows the base peak chromatogram of the xylem sap. Figure 4: Detection of root-derived [Ara 3 ]CLE-RS2 peptide in shoot xylem sap. ( a ) Nano-LC-MS chromatogram of shoot xylem sap collected from soybean plants, in which CLE-RS2 is overexpressed in transformed hairy roots. Selected ion chromatogram at m/z 908.9 that corresponds to [M+2H] 2+ showed a peak at 34.8 min. Inset shows the base peak chromatogram of shoot xylem sap. ( b ) Nano-LC-MS chromatogram of shoot xylem sap collected from soybean transformed with an empty vector. Selected ion chromatogram at m/z 908.9 indicates the absence of [Ara 3 ]CLE-RS2. ( c ) MS/MS spectrum of the 34.8 min peak in a showed a fragmentation pattern identical to that of authentic [Ara 3 ]CLE-RS2. ( d ) Nano-LC-MS chromatogram of shoot xylem sap collected from soybean plants that developed transformed hairy roots after inoculation with a vector harbouring the CLE-RS2 genomic region. Selected ion chromatogram at m/z 606.3 that corresponds to [M+3H] 3+ showed a peak at 35.8 min. Inset shows the base peak chromatogram of the xylem sap. Full size image To eliminate the possibility that [Ara 3 ]CLE-RS2 in the xylem sap is due to unnatural leakage from tissues following its overexpression, we tested whether [Ara 3 ]CLE-RS2 could be detected in xylem sap when CLE-RS2 was driven by its own promoter. We transfected a genomic fragment of CLE-RS2 containing 3.2 kb upstream and 1.2 kb downstream regions from the open reading frame using the soybean hairy root system. The plants were inoculated with rhizobia, and 3 days after inoculation xylem sap was collected from the shoots. Partially purified xylem sap was directly analysed by nano-LC-MS. We confirmed that the selected ion chromatogram for m / z 606.3, which corresponds to [M+3H] 3+ of [Ara 3 ]CLE-RS2, showed a detectable peak at 35.8 min ( Fig. 4d ). Thus, [Ara 3 ]CLE-RS2 was loaded into xylem sap under native expression levels. On the other hand, mass peaks corresponding to possible endogenous soybean CLE peptides were not detected in the partially purified xylem sap. Peptide recovery rate from xylem sap by o -chlorophenol extraction and peptide ionization efficiency by mass spectrometry are often affected by their amino-acid sequences [24] . Soybean CLE peptides, similar in structure to L. japonicus CLE-RS2 but with several amino-acid substitutions, might have lost in these steps. In conclusion, these results indicate that root-derived [Ara 3 ]CLE-RS2 is transported from the root to the shoot through the xylem. Although the existence of a root-derived signal (also known as ‘Q’) was first proposed more than 20 years ago, it has long escaped identification [5] . A possible involvement of secreted peptides in autoregulation of nodulation was first suggested by identification of CLV1-like receptor kinase HAR1, and subsequently supported by identification of root-expressed CLE-RS peptide genes in L. japonicus that act upstream of HAR1. In contrast to the other known Arabidopsis CLE peptides, however, commercially available synthetic CLE domain peptides of CLE-RS family showed no biological activities [16] . Thus, until now, it was not clear whether CLE-RS peptides indeed act as ascending mobile signals that directly interact with HAR1. In this paper, we determined that the mature form of CLE-RS2 is a post-translationally arabinosylated 13-amino-acid glycopeptide derived from the conserved C-terminal CLE domain. Arabinosylated CLE-RS peptides directly bound to HAR1 receptor kinase and showed strong biological activity to suppress nodulation at nanomolar concentrations when applied to shoots. In addition, [Ara 3 ]CLE-RS2 glycopeptide specifically expressed in the root can be detected in xylem sap collected from the shoot. Overall, our findings strongly suggest that arabinosylated CLE-RS peptides are the long sought root-derived signals involved in autoregulation of nodulation. Our analyses showed that arabinosylation of CLE-RS1 and CLE-RS2 is critical for HAR1 binding and activation. This finding further supports the physiological importance of Hyp-arabinosylation in peptide signalling. Initial studies in Arabidopsis reported that arabinosylation of CLV3 glycopeptide considerably enhances its binding to CLV1 receptor kinase [26] . A recent conformational analysis of [Ara 3 ]CLV3 showed that the arabinose chain of [Ara 3 ]CLV3 extends towards the C-terminal end of the peptide and causes distinct distortion in the C-terminal half of the peptide in a highly directional manner [27] . In this context, the arabinose chain of CLE-RS peptides is likely to have a role in maintaining a specific conformation of the peptide backbone rather than directly interacting with receptors. This speculation is supported by our observation that, despite the presence of the arabinose chain, [Ara 3 ]CLV3 did not bind to HAR1. Xylem primarily transports mineral-containing water from the soil to the aerial plant parts. However, we show here that the xylem also transports peptide signals that mediate systemic responses in plants. It remains to be elucidated whether the xylem loading of [Ara 3 ]CLE-RS2 glycopeptide is a passive (non-selective) or an active (selective) process; however, some known xylem proteins appear to be specifically expressed in roots suggesting the presence of a system for secretion into the xylem from the root cells [30] , [31] . How [Ara 3 ]CLE-RS2 glycopeptide is loaded into root xylem is a topic of great interest for future study. The increased understanding of peptide signalling over the last two decades has established that secreted peptides principally have roles in local cell-to-cell communication within specific tissues in plants [32] . In this study, we provide the first indication that a secreted peptide ligand and a receptor kinase mediate long-distance organ-to-organ signalling that leads to a whole-plant systemic response. Although autoregulation of nodulation is a mechanism particularly associated with legumes, organ-to-organ communication is undoubtedly essential in all plant species for coordinated growth and for adaptation to environmental stresses at the whole-plant level [33] , [34] . Additionally, the fact that a large number of secreted peptide genes in the plant genome remain to be characterized, suggests that peptide signalling in plants might prove to be much more dynamic and diverse than previously anticipated. Extraction of secreted peptides Arabidopsis thaliana clv1-1 mutants were transformed using Agrobacterium tumefaciens GV3101, which harbours a p35S : CLE-RS2 construct [16] , via the floral dip method [35] . Transformants were selected using 20 μg ml −1 hygromycin. The resulting T3 plants (10 days after germination, DAG) were subjected to whole-plant submerged culture in 200 ml medium [24] . Secreted peptides accumulating after 24 days of culture were extracted by o -chlorophenol and fractionated in a gel-filtration column [24] , [26] . Transformed hairy roots were induced by infecting L. japonicus B-129 Gifu with Agrobacterium rhizogenes AR1193 harbouring a p35S : CLE-RS2 construct [16] . At 10–14 days after infection, green fluorescent protein-positive hairy roots were selected and cultured for a month in 100 ml of B5 medium containing 1.0% sucrose; the cultures were maintained in the dark at 24 °C with shaking at 100 r.p.m. The medium was then replaced with B5 medium containing 1.0% sucrose and 25 mM CaCl 2 , and the culture continued for 2 weeks without shaking. Secreted peptides that accumulated in the culture medium (200 ml) were extracted and fractionated as above. Nano-LC-MS and nano LC-MS/MS analyses Nano-LC-MS analysis was performed using a DiNa-M splitless nano-HPLC system (KYA Technologies) connected to an LTQ Orbitrap XL mass spectrometer (Thermo Fisher Scientific). Aliquots of apoplastic small peptide fractions (5–10 μl) were loaded onto a trap column (0.5 mm i.d. × 1 mm cartridge, C18; KYA Technologies) and washed with 0.1% formic acid. Peptides were subsequently eluted from the precolumn and separated on a long nano-column (100 μm i.d. × 750 mm, MonoCap C18 High Resolution 750; GL Sciences), with a gradient of 2–50% acetonitrile (containing 0.1% formic acid) for 90 min at a flow rate of 500 nl min −1 . The nano-HPLC eluate was introduced into a mass spectrometer via an electrospray ionization (ESI) interface at a spray voltage of 2.0 kV. The mass spectrometer was operated in positive ion mode with a capillary temperature of 160 °C. Mass spectra were obtained by scanning from m/z 400 to m/z 1,500. Nano-LC-MS/MS analysis was performed in manual scan mode, selecting the indicated molecular ion as the precursor ion at 30% normalized collision energy using the higher energy collision dissociation mode. Synthesis of [Ara 3 ]CLE-RS peptides Asp( t Bu)-Pro-Gln(Trt)-His(Trt)-Asn(Trt)-Asn(Trt)-resin was prepared by conventional solid-phase peptide synthesis using an ABI 431A peptide synthesizer. A mixture of Fmoc-[AcAra 3 ]Hyp-OH (6.0 mg, 5.8 μmol) [27] , 1-hydroxybenzotriazole (2.7 mg, 20 μmol), O -benzotriazole- N,N,N′,N′ -tetramethyluronium hexafluorophosphate (7.6 mg, 20 μmol) and N,N -diisopropylethylamine (7.0 μl, 40 μmol) dissolved in dry N -methylpyrrolidone (200 μl) was added to the peptide-resin (25 μmol) pre-swollen with dry N -methylpyrrolidone (50 μl). The mixture was stirred for 2 h at room temperature. Peptide-resin was recovered by filtration, and the remaining N-terminal amino acids were added to the peptide using the peptide synthesizer. The synthesized peptide was deprotected and cleaved from the resin using trifluoroacetic acid/water (95:5 v/v, 1 ml) for 30 min and then precipitated using ether (10ml) at −20 °C for 5 min. The precipitated peptide was washed twice with cold ether, dissolved in water and lyophilized. Crude peptide was dissolved in dry methanol (3 ml) and treated with sodium methoxide (28% solution, 60 μl) at room temperature for 1 h. The reaction was terminated by adding acetic acid (60 μl). HPLC purification using an amide column (TSK-gel amide-80, TOSOH) gave analytically pure [Ara 3 ]CLE-RS2 (1.5 mg). For the synthesis of [Ara 3 ]CLE-RS1 glycopeptide, Asp( t Bu)-Pro-Gln(Trt)-His(Trt)-Asn(Trt)-Gly-resin was used as the starting material. Bioassay Sterilized seeds of L. japonicus B-129 Gifu (wild type) or the hypernodulating mutant har1-4 ( sym78-1 ) were germinated and grown in plastic boxes with sterilized vermiculite moistened with liquid Broughton and Dilworth (B&D) medium in a growth cabinet (22 °C, 16 h light/22 °C, 8 h dark). At 6 DAG, the distal half of each cotyledon was excised and the remaining half was inserted into a plastic tube filled with peptide solution. Next day, plants were inoculated with M. loti MAFF303099 and were grown for a further 14 days. The peptide solution was supplemented every 3 days to ensure continuous immersion of the cut cotyledon surface. Nodule numbers were counted at 14 days after inoculation. The effectiveness of the technique was confirmed using uptake of blue dye (Palace Chemicals, Japan) into primary shoot leaves. Synthesis of photoactivatable ASA-[Ara 3 ]CLE-RS2 The Fmoc-protected [Ara 3 ]CLE-RS2 analogue, Fmoc-[Lys 2 ][Ara 3 ]CLE-RS2, was synthesized as described above. 4-Azidosalicylic acid succinimidyl ester (0.2 mg, Pearce), Fmoc-[Lys 2 ][Ara 3 ]CLE-RS2 (1.4 mg) and NaHCO 3 (1.0 mg) were dissolved in 100 μl of 50% acetonitrile and stirred for 2 h in the dark at room temperature. Crude peptide was purified by reverse-phase HPLC and lyophilized to yield Fmoc-[(4-azidosalicyl)Lys 2 ][Ara 3 ]CLE-RS2; 50 μl of 50% piperidine in acetonitrile was added to the purified peptide, followed by incubation for 1 h in the dark at room temperature. The deprotected peptide was further purified by reverse-phase HPLC and lyophilized to obtain analytically pure [(4-azidosalicyl)Lys 2 ][Ara 3 ]CLE-RS2 (ASA-[Ara 3 ]CLE-RS2) (0.34 mg). ASA-[Ara 3 ]CLE-RS2 was radioiodinated using the chloramine T method [36] . Labelled peptide was purified by reverse-phase HPLC to yield analytically pure [ 125 I]ASA-[Ara 3 ]CLE-RS2 with a specific radioactivity of 85 Ci mmol −1 . Expression of HAR1–HT and photoaffinity labelling To overexpress HAR1–HT in tobacco BY-2 cells, we PCR amplified the genomic fragment of HAR1 corresponding to the Met 1 to Glu 702 region, and the cDNA fragment of HaloTag (Promega) containing the entire open reading frame of HaloTag. The two fragments were cloned in translational fusion by three-component ligation into the BamHI/SacI-digested binary vector pBI121 using an In-Fusion HD Cloning Kit (Clontech). To prepare HAR1 L246F -HT, the amino-acid substitution L246F was introduced into HAR1–HT by PCR-based site-directed mutagenesis. Transformation of tobacco BY-2 cells and preparation of microsomal fractions were described previously [36] . To confirm expression, HaloTag-fused proteins were specifically labelled using HaloTag TMR (Promega), separated by SDS–polyacrylamide gel electrophoresis, and visualized by a fluorescent image analyzer with a 523 nm excitation filter and a 580 nm emission filter. Photoaffinity labelling was performed as described [28] . Hairy root transformation and collection of xylem sap G. max Enrei seedlings (5 DAG) were inoculated with A. rhizogenes K599 harbouring either a CLE-RS2 -overexpressing construct or an empty vector. Hairy root transformation was induced [37] , and the plants were grown on vermiculite. Three weeks after inoculation, untransformed roots were removed, and plants with green fluorescent protein-positive hairy roots were transplanted into fresh sterilized vermiculite. Three weeks after replanting, the stem was cut at the second internode above the hypocotyl and xylem sap was collected. Approximately 30 ml xylem sap was obtained from 4 CLE-RS2 -overexpressing plants, and almost same amount of xylem sap was obtained from five plants transformed with an empty vector. Peptides in the xylem sap were extracted, size-fractionated and subjected to nano-LC-MS and nano-LC-MS/MS analyses as above. To express CLE-RS2 under the control of its own promoter, a genomic fragment of CLE-RS2 containing an approximately 3.2 kb upstream region and a 1.2 kb downstream region from the open reading frame was cloned using the primers 5′-AGGCTTTAACTCATTGCATC-3′ and 5′-ATTGCACAGTAATGGTTTCC-3′. Hairy root transformation was performed as above. Three weeks after replanting, the plants were inoculated with Bradirhizobium japonicum A1017; after 3 days, 1.5 ml xylem sap was obtained from each plant. Peptides in the xylem sap were extracted by o -chlorophenol and subjected to nano-LC-MS and nano-LC-MS/MS analyses as above. How to cite this article: Okamoto, S. et al . Root-derived CLE glycopeptides control nodulation by direct binding to HAR1 receptor kinase. Nat. Commun. 4:2191 doi: 10.1038/ncomms3191 (2013).